GATA-dependent regulatory switches establish atrioventricular canal specificity during heart development The embryonic vertebrate heart tube develops an atrioventricular canal that divides the atrial and ventricular chambers, forms atrioventricular conduction tissue and organizes valve development. Here we assess the transcriptional mechanism underlying this localized differentiation process. We show that atrioventricular canal-specific enhancers are GATA-binding site-dependent and act as switches that repress gene activity in the chambers. We find that atrioventricular canal-specific gene loci are enriched in H3K27ac, a marker of active enhancers, in atrioventricular canal tissue and depleted in H3K27ac in chamber tissue. In the atrioventricular canal, Gata4 activates the enhancers in synergy with Bmp2/Smad signalling, leading to H3K27 acetylation. In contrast, in chambers, Gata4 cooperates with pan-cardiac Hdac1 and Hdac2 and chamber-specific Hey1 and Hey2, leading to H3K27 deacetylation and repression. We conclude that atrioventricular canal-specific enhancers are platforms integrating cardiac transcription factors, broadly active histone modification enzymes and localized co-factors to drive atrioventricular canal-specific gene activity. Congenital heart defects affect ~1% of live births, and are found in up to 10% of spontaneously aborted fetuses [1] . Better insight into the transcriptional networks governing heart development would help to shed light on the origin and aetiology of congenital heart defects. A highly conserved step in the evolution of vertebrates is the division of the heart in atrial and ventricular chambers by the atrioventricular (AV) canal [2] . This step is crucial for heart structure and pump function. Defects in AV canal development account for a large fraction of congenital heart defects [3] , [4] , [5] . The initially formed heart tube consists of embryonic myocardium that proliferates slowly and conducts the electrical impulse at a slow rate [6] . While the tube elongates, specific regions differentiate and start to proliferate to form the expanding atria and ventricles. In contrast, the region in between the atrial and ventricular chambers does not expand but forms the AV canal. The cells of the AV canal preserve characteristics of the embryonic myocardium. The AV canal is required for septation and valve formation [7] , and forms pacemaker tissues that slowly conduct the impulse from atria to ventricles ensuring their sequential contraction [6] . During development, embryonic myocardial cells are thus confronted with a critical decision: differentiation into pacemaker-like cardiomyocytes of the AV canal or into working cardiomyocytes of the atrial and ventricular chambers. This decision is, at least in part, imposed by Bmp2-mediated signalling and the T-box transcription factors Tbx2 and Tbx3, which are selectively active in the AV canal where they suppress a default chamber gene programme [8] , [9] , [10] . However, how AV canal-specific gene expression is regulated is not understood. An enhancer upstream of chicken Gata6 directs transgene expression throughout the primary heart tube and at later stages in the AV canal [11] , [12] . Furthermore, enhancers of Tbx2 (ref. 13 ) and Gjd3 (Cx30.2) [14] and the promoter of Tnni3 (cTnI) [15] confer AV canal-restricted gene activity in transgenic mouse embryos. Tbx2 was found to be activated by Bmp-signalling mediating Smads [13] , whereas the activity of the Cx30.2 enhancer depends on the broadly expressed factors Tbx5 and Gata4 (ref. 14 ). Nevertheless, the mechanism for the AV canal specificity has remained unclear. Here, we investigated the regulatory mechanism underlying the AV canal-specific activity of these enhancers. We describe a mechanism by which GATA-dependent AV canal-specific enhancers mediate tissue-dependent gene activation and repression. GATA-binding elements in such enhancers recruit a Gata4/Smad4/HAT transcriptional activation complex in the AV canal and a Gata4/Hey1, 2/HDAC transcriptional repression complex in the chambers. The former induces H3K27 acetylation that is associated with AV canal gene activation, the latter induces H3K27 deacetylation associated with repression of AV canal genes in the chamber myocardium. GATA-dependent AV canal enhancers act as chamber repressors We first tested whether a mechanism of repression could be involved in the restriction of the activity of AV canal-specific enhancers to the AV canal. The promoter of the rat cardiac troponin T (cTnT, Tnnt2) gene drives efficient pan-cardiac expression in transgenic mice [16] ( Fig. 1a,b ). Previous analysis revealed that a tandem array of four copies of a 102 bp (−1420/−1319) cGata6 enhancer module recapitulates AV canal specificity [12] . This tandem array was coupled to the cTnT promoter and the activity was assayed in E11.5 transgenic embryos. Strikingly, the cGata6 module restricts activity of the cTnT-lacZ transgene construct to the AV canal, indicating that it acts as repressor of the cTnT promoter in the chambers ( Fig. 1c,d ). The cGata6 module does not appear to be conserved in mammals. Therefore, we next tested the conserved AV canal-specific mouse Tbx2 enhancer [13] . An array of four copies of the 380 bp enhancer likewise restricted cTnT -driven expression to the AV canal ( Fig. 1e,f ), indicating this was not a specific property of the cGata6 module, but a general property of AV canal-specific enhancers. We conclude that these AV canal enhancers act as tissue-specific switches, activating gene expression in the AV canal and repressing gene expression in the chambers. 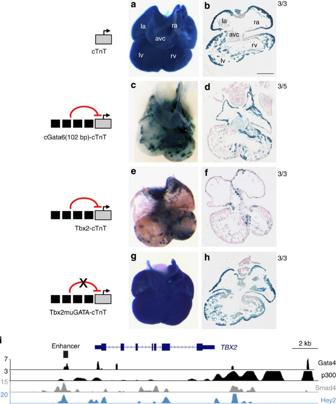Figure 1: GATA sites are required to mediate repression of AV canal genes in chamber myocardium. Localization of transgene expression in E11.5 mouse hearts. (a,b) ThecTnTtransgene is expressed both in the AV canal myocardium and the chamber myocardium. (c,d)cGata6-cTnTtransgenics show predominant expression in the AV canal, similar to the pattern of theTbx2-cTnTtransgenes (e,f). (g,h) Mutation of the two GATA sites in theTbx2regulatory region removes the repression in the chambers. Ratios denote proportion of embryos showing chamber repression. Scale bar represents 100 μm. (la) left atrium; (ra) right atrium; (avc) AV canal; (lv) left ventricle; (rv) right ventricle; (oft) outflow tract. (i) Browser view ofTbx2gene locus with ChIP-seq profiles of Gata4 (ref.18) (black) and p300 (ref.24) (black) in heart, Smad4 (grey) in human ESC31and Hey2 (blue) in mouse ESC. The 380 bpTbx2(−2700/−2300) enhancer region is depicted as a black box. Figure 1: GATA sites are required to mediate repression of AV canal genes in chamber myocardium. Localization of transgene expression in E11.5 mouse hearts. ( a , b ) The cTnT transgene is expressed both in the AV canal myocardium and the chamber myocardium. ( c , d ) cGata6-cTnT transgenics show predominant expression in the AV canal, similar to the pattern of the Tbx2-cTnT transgenes ( e , f ). ( g , h ) Mutation of the two GATA sites in the Tbx2 regulatory region removes the repression in the chambers. Ratios denote proportion of embryos showing chamber repression. Scale bar represents 100 μm. (la) left atrium; (ra) right atrium; (avc) AV canal; (lv) left ventricle; (rv) right ventricle; (oft) outflow tract. ( i ) Browser view of Tbx2 gene locus with ChIP-seq profiles of Gata4 (ref. 18 ) (black) and p300 (ref. 24 ) (black) in heart, Smad4 (grey) in human ESC [31] and Hey2 (blue) in mouse ESC. The 380 bp Tbx2 (−2700/−2300) enhancer region is depicted as a black box. Full size image The AV canal-specific enhancers of cGata6 , Cx30.2 , Tbx2 and promoter of cTnI contain GATA-binding sites [12] , [13] , [14] , [17] ( Supplementary Fig. 1 ). Gata4 chromatin immunoprecipitation (ChIP)-sequence data from adult hearts [18] revealed that Gata4 binds the AV canal-specific regulatory elements in vivo ( Fig. 1i ). This was confirmed by chromatin immunoprecipitation quantitative polymerase chain reaction using extracts prepared form AV canal or from the chambers ( Supplementary Figs 2,3b ). To assess whether the GATA sites are required for AV canal activity, we made use of a mouse heart organ culture and transfection assay to measure enhancer activities. We observed that mutation of the GATA-binding sites affected the activation of both the cGata6 and Tbx2 enhancer in AV canal explants ( Supplementary Fig. 3d ). Next, the GATA-binding sites were mutated in the cTnT promoter-coupled Tbx2 enhancer. We observed loss of repression of the cTnT promoter in the chambers in vivo ( Fig. 1g,h ). These data revealed that the GATA sites are required for the repressive activity of this enhancer. To identify additional binding elements involved in the activity of AV canal enhancers, we contrasted Gata4 ChIP sequencing data [18] and a set of AV canal-enriched genes [19] . This analysis indicated that Gata4-binding sites close to or in AV canal-enriched genes are often associated with the presence of the binding site motif for the Sp family of transcription factors ( Supplementary Fig. 4a ). The 47 bp core module of the cGata6 enhancer [12] that contains a Sp-binding motif was mutated to only preserve the GATA-binding sites (cGata6muSP(GATA) 2 ). Eight copies of the mutated module (cGata6muSP(GATA) 16 ) were coupled to the cTnT-promoter lacZ reporter. We found that the ability of the module with the mutated Sp site to repress transcription in the chamber myocardium was preserved, but with lower efficiency ( Supplementary Fig. 4c ). We conclude that the GATA sites are sufficient to mediate transcriptional repression in chamber myocardium. Assessment of H3K27 acetylation in AV canal and chambers Gata4 itself is not localized, but is present in the nuclei of both AV canal and chamber myocardium in identical subnuclear localization patterns ( Supplementary Fig. 3c ). Therefore, we speculated that Gata4 cooperates with a localized factor that mediates gene activation in the AV canal or gene repression in the chambers. Previous work identified Gata4 as a regulator of histone modifications by physically interacting with Hats and Hdacs [20] . Therefore, we tested whether AV canal-specific enhancers are differentially marked by acetylation of histone H3 lysine 27, a modification associated with active enhancers and with Hat p300 activity [21] , [22] . To this end, the genome-wide distribution of H3K27ac was assessed by ChIP-seq of purified embryonic AV canal cells and of chamber cells. We generated E10.5 double transgenic embryos in which the expression of the green fluorescent protein (EGFP) (Tbx3BAC-GFP [19] ) is restricted to the AV canal and of the red fluorescent protein Katushka (NppbBAC-Katushka [23] ) is restricted to the chamber myocardium ( Fig. 2a,b ). EGFP and Katushka-positive cells were purified by fluorescence-activated cell sorting ( Fig. 2c , Supplementary Fig. 5 ) and used for ChIP-seq ( Fig. 2e ). We asked whether DNA regions differentially enriched between the AV canal and chambers for H3K27ac were selectively associated with genes specifically expressed in the AV canal that were previously identified [19] ( Supplementary Tables 1,2 ). The loci of the 50 genes whose expression is most significantly enriched in embryonic AV canal were also significantly enriched in AV canal-specific H3K27ac marks, indicating that activity in the AV canal is associated with H3K27 acetylation. The enrichment was validated in a small set of genes whose specific expression in AV canal myocardium has been established ( Cacna1g , Cacna2d2 , Kcna6 , Msx2 , Tbx2 , Tbx3 , Id1 , Id2, Gjd3, Robo1 and Bmp2, Supplementary Tables 1,2 ). Furthermore, H3K27ac marks in loci harbouring genes expressed in both AV canal and chambers (including Gata4 , Gata6 , Nkx2-5 , Tbx5 , etc.) were distributed equally between AV canal and chambers. Chamber-specific H3K27ac marks were enriched in a set of chamber-specific gene loci ( Hey2 , Nppa , Nppb , Fig. 2e and ChIP-seq data set). This was confirmed by chromatin immunoprecipitation quantitative polymerase chain reaction from purified AV canal and chamber cells ( Fig. 2f ). For broadly expressed genes such as Gata4, our ChIP-seq data correlated with the H3K27ac E14.5 heart data of ENCODE [24] ( Fig. 2e ), whereas AV canal-specific H3K27ac signals were nearly undetectable in the ENCODE set as expected ( Fig. 2e ; E14.5 whole heart is composed of a very small fraction AV canal). 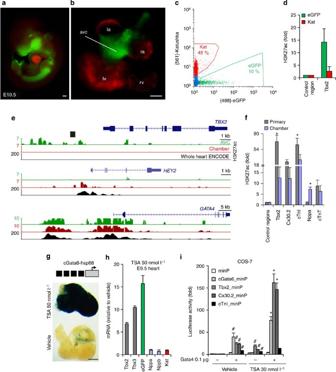Figure 2: Repression of GATA-dependent AV canal enhancers in chamber myocardium is mediated by Hdacs and deacetylation of histone H3K27. Whole-mount fluorescence microscopy of double transgenic E10.5 embryo (a) and E10.5 heart (b). (c) Fluorescence-activated cell sorting profile of double AV canal-EGFPand chambers–Katushka transgenic E10.5 hearts. Scale bars represent 100 μm. (d) Chromatin immunoprecipitation quantitative polymerase chain reaction (ChIP–qPCR) assay with H3K27ac antibody using EGFP and Kat sorted cells. Bars represent mean±s.d. (n=3). (e) Alignment of H3K27a ChIP-seq profiles from EGFP (green), Kat (red) sorted cells and E14.5 whole hearts24(black). (f) ChIP–qPCR assay with H3K27ac antibody using dissected AV canal/outflow tract and chamber myocardium extracts. Bars represent mean±s.e.m. (n=3). Statistical test was conducted using the Student’s two-tailedt-test (*P<0.05). (g) E10.5cGata6-hsp68transgenic hearts were cultured in the presence or absence of 50 nmol l−1TSA for 48 h. TSA-treated littermate hearts displayed pan-myocardiallacZexpression. In control medium, the reporter gene remained confined to the AV canal. Scale bar represents 100 μm. (h) E9.5 chambers–Katushka/AV canal-EGFP transgenic hearts were cultured in the presence or absence of 50 nmol l−1TSA for 48 h, and expression of AV (Tbx2, Tbx3, EGFP) and chamber markers (Nppa, Nppb, Katushka) was analysed with real time RT–PCR. Data were normalized toHPRTand expressed as folds of increase over untreated samples. (i) Luciferase reporter assays on 102 bpcGata6, the 380 bpTbx2, 660 bpCx30.2and the 356 bpcTnIgenomic fragments. Cos-7 cells co-transfected with Gata4 expressing vector or not were treated in the absence or presence of 30 nmol l−1TSA. Bars represent mean±s.e.m. (n=6). Statistical test was conducted using the two- and three-way analysis of variance (#P<0.05 for Gata4 or TSA treatment versus control, *P<0.05 for Gata4 and TSA treatment versus Gata4 or TSA treatment). Figure 2: Repression of GATA-dependent AV canal enhancers in chamber myocardium is mediated by Hdacs and deacetylation of histone H3K27. Whole-mount fluorescence microscopy of double transgenic E10.5 embryo ( a ) and E10.5 heart ( b ). ( c ) Fluorescence-activated cell sorting profile of double AV canal- EGFP and chambers–Katushka transgenic E10.5 hearts. Scale bars represent 100 μm. ( d ) Chromatin immunoprecipitation quantitative polymerase chain reaction (ChIP–qPCR) assay with H3K27ac antibody using EGFP and Kat sorted cells. Bars represent mean±s.d. ( n =3). ( e ) Alignment of H3K27a ChIP-seq profiles from EGFP (green), Kat (red) sorted cells and E14.5 whole hearts [24] (black). ( f ) ChIP–qPCR assay with H3K27ac antibody using dissected AV canal/outflow tract and chamber myocardium extracts. Bars represent mean±s.e.m. ( n =3). Statistical test was conducted using the Student’s two-tailed t -test (* P <0.05). ( g ) E10.5 cGata6-hsp68 transgenic hearts were cultured in the presence or absence of 50 nmol l −1 TSA for 48 h. TSA-treated littermate hearts displayed pan-myocardial lacZ expression. In control medium, the reporter gene remained confined to the AV canal. Scale bar represents 100 μm. ( h ) E9.5 chambers–Katushka/AV canal-EGFP transgenic hearts were cultured in the presence or absence of 50 nmol l −1 TSA for 48 h, and expression of AV ( Tbx2, Tbx3, EGFP ) and chamber markers ( Nppa, Nppb, Katushka ) was analysed with real time RT–PCR. Data were normalized to HPRT and expressed as folds of increase over untreated samples. ( i ) Luciferase reporter assays on 102 bp cGata6 , the 380 bp Tbx2 , 660 bp Cx30.2 and the 356 bp cTnI genomic fragments. Cos-7 cells co-transfected with Gata4 expressing vector or not were treated in the absence or presence of 30 nmol l −1 TSA. Bars represent mean±s.e.m. ( n =6). Statistical test was conducted using the two- and three-way analysis of variance ( # P <0.05 for Gata4 or TSA treatment versus control, * P <0.05 for Gata4 and TSA treatment versus Gata4 or TSA treatment). Full size image The occupancy profile of Gata4 colocalized with regional H3K27 acetylation on AV canal enhancers ( Fig. 1i , Supplementary Fig. 2 ). 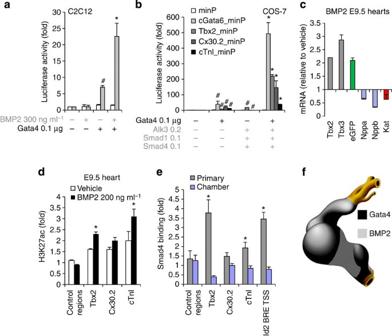Figure 3: The Gata4-Smad-Hat complex induces H3K27 acetylation and AV canal gene activation. (a) Luciferase reporter assays on the 102 bpcGata6enhancer. Plasmids encoding full-length Gata4 protein, the luciferase reporter construct with a minimal promoter (minP) or containing thecGata6enhancer with the same minimal promoter (cGata6_minP) were co-transfected in C2C12 cells. The cells were incubated with or without the recombinant human BMP2. Statistical test was conducted using two- and three-way analysis of variance (ANOVA) (mean±s.e.m.,n=3,#P<0.05 for Gata4 or BMP2 treatment versus control, *P<0.05 for Gata4 and BMP2 treatment versus Gata4 or BMP2 treatment). (b) Luciferase reporter assays on the 102 bpcGata6, the 380 bpTbx2, 660 bpCx30.2and the 356 bpcTnIgenomic fragments. Constructs were co-transfected with Gata4, Alk3CA, Smad1 and Smad4 expression vectors into Cos-7 cells. Luciferase activity was determined and normalized as fold over the reporter alone (mean±s.e.m.,n=6,#P<0.05 for Gata4 or BMP2 effectors versus control, *P<0.05 for Gata4 and BMP2 effectors versus Gata4 or BMP2 effectors, using two- and three-way ANOVA). (c) E9.5 chambers–Katushka/AV canal-EGFP transgenic hearts were cultured in the presence or absence of 200 ng ml−1Bmp2 for 48 h, and expression of AV canal (Tbx2, Tbx3, EGFP) and chamber markers (Nppa, Nppb, Kat) was analysed with real time RT–PCR. Data were normalized toHPRTand expressed as folds of increase over untreated samples. (d) Untreated and Bmp2-treated E9.5 hearts were subjected to ChIP assay analyses with anti-H3K27ac antibody. Histograms represent enrichment forTbx2,Cx30.2andcTnIregulatory enhancers (mean±s.e.m.,n=3, *P<0.05 using the Student’s two-tailedt-test). (e) ChIP–qPCR analysis with Smad4 antibody on E10.5 embryo extracts from AV canal/outflow tract and chamber myocardium. Primers amplifying the BRE of theId2promoter serve as a positive ChIP control27. Pulled-down DNA fragments were analysed with real-time PCR and enrichment indicates the ratio of ChIPed DNA to negative control regions, normalized for input DNA (mean±s.e.m.,n=3, *P<0.05 using the Student’s two-tailedt-test). (f) Cartoon depicting the overlapping expression patterns of Bmp2/Smad4 and Gata4 at stage E9.5–E10.5. Gene ontology analysis of the gene sets co-occupied by Gata4 and either AV canal-specific H3K27ac or chamber-specific H3K27ac revealed that both sets were enriched for terms related to heart development ( Supplementary Table 3 ). The Gata4-AV canal-specific H3K27ac set was enriched for terms related to cell metabolism. In contrast, the Gata4-chamber-specific H3K27ac set was enriched in genes linked to muscle differentiation and muscle cytoskeleton organization, which is in line with the notion that chamber myocytes acquire more mature cardiac muscle properties compared with the AV canal myocytes. These data indicate that in the two compartments different gene loci are both occupied by Gata4 and marked by H3K27ac. To assess whether the repression of AV canal enhancers in chamber myocardium is mediated by Hdac-mediated deacetylation, explanted embryonic mouse hearts of the cGata6-lacZ line were treated with trichostatin-A (TSA) that blocks Hdac activity [25] . When cultured in control medium, the reporter gene remained confined to the AV canal whereas TSA-treated littermate hearts displayed pan-myocardial lacZ expression ( Fig. 2e ). Expression of AV canal-specific Tbx2 , Tbx3 and EGFP driven by Tbx3 regulatory regions [19] increased in explanted E9.5 embryonic hearts treated with TSA compared with dimethylsulphoxide-treated explants ( Fig. 2h ). We next assessed the activity of the 380 bp Tbx2 enhancer, the 660 bp Cx30.2 enhancer and the 356 bp cTnI promoter in TSA-treated cells ( Fig. 2i ). Inhibition of Hdacs increased the luciferase activity of the reporter constructs ( Fig. 2i ). These enhancers were synergistically and strongly induced by the combination of both TSA and Gata4. Smad4 and Gata4 cooperatively mediate H3K27ac Bmp2 signalling is selectively active in the AV canal myocardium [26] . Its downstream effector Smad4 can physically interact with Gata4 [27] and recruit the histone acetyltransferase p300 to specific chromatin loci [28] , [29] , [30] . We evaluated the transcriptional regulation of AV canal enhancers by Gata4 and Bmp2 signalling. The cGata6 enhancer (three tandem copies) showed a 7-fold activation by Gata4 in mouse C2C12 myoblast cells ( Fig. 3a ). The enhancer was not activated by Bmp2 alone, but was synergistically induced about 25-fold by the combination of Bmp2 and Gata4. The 380 bp Tbx2 enhancer, the 660 bp Cx30.2 enhancer and the 356 bp cTnI promoter were moderately induced by either Bmp effectors alone (constitutive active Alk3, Smad1 and Smad4) or Gata4 alone. In contrast, co-transfection of both Bmp effectors and Gata4 produced a very strong synergistic induction in reporter activity ( Fig. 3b ). Figure 3: The Gata4-Smad-Hat complex induces H3K27 acetylation and AV canal gene activation. ( a ) Luciferase reporter assays on the 102 bp cGata6 enhancer. Plasmids encoding full-length Gata4 protein, the luciferase reporter construct with a minimal promoter (minP) or containing the cGata6 enhancer with the same minimal promoter ( cGata6_minP ) were co-transfected in C2C12 cells. The cells were incubated with or without the recombinant human BMP2. Statistical test was conducted using two- and three-way analysis of variance (ANOVA) (mean±s.e.m., n =3, # P <0.05 for Gata4 or BMP2 treatment versus control, * P <0.05 for Gata4 and BMP2 treatment versus Gata4 or BMP2 treatment). ( b ) Luciferase reporter assays on the 102 bp cGata6 , the 380 bp Tbx2 , 660 bp Cx30.2 and the 356 bp cTnI genomic fragments. Constructs were co-transfected with Gata4, Alk3CA, Smad1 and Smad4 expression vectors into Cos-7 cells. Luciferase activity was determined and normalized as fold over the reporter alone (mean±s.e.m., n =6, # P <0.05 for Gata4 or BMP2 effectors versus control, * P <0.05 for Gata4 and BMP2 effectors versus Gata4 or BMP2 effectors, using two- and three-way ANOVA). ( c ) E9.5 chambers–Katushka/AV canal-EGFP transgenic hearts were cultured in the presence or absence of 200 ng ml −1 Bmp2 for 48 h, and expression of AV canal ( Tbx2, Tbx3, EGFP ) and chamber markers ( Nppa, Nppb, Kat ) was analysed with real time RT–PCR. Data were normalized to HPRT and expressed as folds of increase over untreated samples. ( d ) Untreated and Bmp2-treated E9.5 hearts were subjected to ChIP assay analyses with anti-H3K27ac antibody. Histograms represent enrichment for Tbx2 , Cx30.2 and cTnI regulatory enhancers (mean±s.e.m., n =3, * P <0.05 using the Student’s two-tailed t -test). ( e ) ChIP–qPCR analysis with Smad4 antibody on E10.5 embryo extracts from AV canal/outflow tract and chamber myocardium. Primers amplifying the BRE of the Id2 promoter serve as a positive ChIP control [27] . Pulled-down DNA fragments were analysed with real-time PCR and enrichment indicates the ratio of ChIPed DNA to negative control regions, normalized for input DNA (mean±s.e.m., n =3, * P <0.05 using the Student’s two-tailed t -test). ( f ) Cartoon depicting the overlapping expression patterns of Bmp2/Smad4 and Gata4 at stage E9.5–E10.5. Full size image Next, in vitro cultured embryonic hearts of the chamber-Katushka/AV canal-EGFP transgenic mouse line ( Fig. 2a,b ) were treated with Bmp2 ( Fig. 3c ), which resulted in induction of endogenous AV canal genes ( Tbx2 , Tbx3 ) and reduction of chamber myocardium markers ( Nppa , Nppb ) ( Fig. 3c ). In vivo ChIP assays demonstrated that the Bmp2-induced gene activity was associated with an enrichment of the activating H3K27ac epigenetic mark on AV canal-specific enhancers ( Fig. 3d ). Analysis of available Smad4 ChIP-seq data [31] from embryonic stem cells (ESC) revealed that Tbx2 , Cx30.2 and cTnI regulatory regions are occupied by Smad4 in this context, suggesting that they can be co-occupied by Smad4 and Gata4 in the heart ( Fig. 1i and Supplementary Fig. 2 ). Smad4 indeed occupies sites also occupied by H3K27ac in E10.5 AV canal myocardium, but not in chamber myocardium ( Fig. 3e ). Consistently, although Smad4 is ubiquitously expressed at E10.5, its localization is predominantly nuclear in the AV canal [32] , [33] . Taken together, the data indicate that AV canal-specific regulatory regions that harbour the GATA elements direct complex formation of Gata4, Smad4 and Hat, implicating these factors in AV canal-specific gene activity in vivo . AV canal enhancers are repressed by Hdacs and Hey1, -2 The AV canal enhancers were associated with H3K27ac in the AV canal, with non-acetylated H3K27 in chamber myocardium, and were activated by TSA treatment. Therefore, we tested whether the transcriptional repression was mediated by Hdacs. Nine Hdac family members are expressed in the developing heart [34] , [35] , [36] . Using real time reverse transcriptase polymerase chain reaction (RT–PCR), we determined their expression levels in the EGFP+ AV canal cells and Katushka+ chamber cells fluorescence-activated cell sorting isolated from E10.5 Tbx3BAC-GFP;NppbBAC-Katushka mouse embryos. None of them was found to be significantly differentially expressed ( Fig. 4b ). We therefore speculated that a locally expressed Gata4 co-repressor might directly or indirectly recruit the broadly expressed Hdacs. Hdac2 can physically interact with Gata4 (ref. 37 ). Furthermore, Hdac1 and 2 are functionally redundant in the heart, and cardiac-specific inactivation of both Hdac1 and 2 resulted in neonatal lethality associated with cardiac arrhythmias [35] . Therefore, we focused on Hdac1 and 2. Both Hdac1 and 2 could prevent the activation of AV canal enhancers by Gata4 and effectors of Bmp2 signalling in cell culture ( Fig. 4a ). Since dynamic changes in the subcellular localization of Hdacs can contribute to gene regulation [38] , we evaluated the subcellular localization of Hdac1 and 2 in E10.5 hearts. Both Hdac1 and 2 were localized in the nucleus in both the AV canal and chamber myocardium ( Fig. 4c,d ). We therefore speculated that a locally expressed Gata4 co-repressor might directly or indirectly recruit the broadly expressed Hdacs. 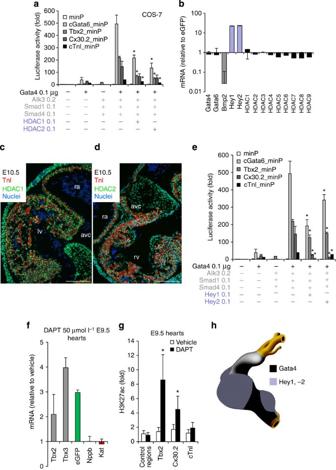Figure 4: The Gata4/Hey/Hdac complex induces H3K27 deacetylation and AV canal gene repression. (a) Luciferase reporter assays on 102 bpcGata6, the 380 bpTbx2, 660 bpCx30.2and the 356 bpcTnIgenomic fragments. Constructs were co-transfected with Gata4, Alk3CA, Smad1 and Smad4, HDAC1 and 2 expression vectors into Cos-7 cells (mean±s.e.m.,n=6, *P<0.05 for Gata4, BMP2 effectors and HDAC1, 2 vs Gata4 and BMP2 co-transfection using two- and three-way analysis of variance (ANOVA)). (b) qPCR analysis of mRNA isolated from AV canal-EGFP and chambers–Katushka sorted cells. Values are normalized againstEGFPpopulation. Immunohistochemistry for Hdac1 (c) and 2 (d) proteins on sections of E10.5 hearts. Scale bars represent 100 μm. (e) Luciferase reporter assays on AV canal enhancers with expressing vectors encoding for Gata4, Bmp2 effectors and the notch target genes Hey1 and 2 (mean±s.e.m.,n=6, *P<0.05 for Gata4, BMP2 effectors and Hey1, 2versusGata4 and BMP2 effectors co-transfection, using two- and three-way ANOVA). (f) E9.5 chambers–Katushka/AV canal-EGFP transgenic hearts were cultured in the presence or absence of 50 μmol l−1γ-secretase inhibitor (DAPT) for 48 h, and expression of AV canal and chamber markers was analysed with real time RT–PCR. Data were normalized toHPRTand expressed as folds of increase over untreated samples. (g) Untreated and DAPT-treated E9.5 hearts were subjected to ChIP assay analyses with anti-H3K27ac antibody. Pulled-down DNA fragments were analysed with RT–PCR and enrichment indicates the ratio of ChIPed DNA to negative control regions, normalized for input DNA. (h) Cartoon depicting the overlapping expressions of Hey1, 2 and Gata4 at stage E9.5–E10.5. Figure 4: The Gata4/Hey/Hdac complex induces H3K27 deacetylation and AV canal gene repression. ( a ) Luciferase reporter assays on 102 bp cGata6 , the 380 bp Tbx2 , 660 bp Cx30.2 and the 356 bp cTnI genomic fragments. Constructs were co-transfected with Gata4, Alk3CA, Smad1 and Smad4, HDAC1 and 2 expression vectors into Cos-7 cells (mean±s.e.m., n =6, * P <0.05 for Gata4, BMP2 effectors and HDAC1, 2 vs Gata4 and BMP2 co-transfection using two- and three-way analysis of variance (ANOVA)). ( b ) qPCR analysis of mRNA isolated from AV canal-EGFP and chambers–Katushka sorted cells. Values are normalized against EGFP population. Immunohistochemistry for Hdac1 ( c ) and 2 ( d ) proteins on sections of E10.5 hearts. Scale bars represent 100 μm. ( e ) Luciferase reporter assays on AV canal enhancers with expressing vectors encoding for Gata4, Bmp2 effectors and the notch target genes Hey1 and 2 (mean±s.e.m., n =6, * P <0.05 for Gata4, BMP2 effectors and Hey1, 2 versus Gata4 and BMP2 effectors co-transfection, using two- and three-way ANOVA). ( f ) E9.5 chambers–Katushka/AV canal-EGFP transgenic hearts were cultured in the presence or absence of 50 μmol l −1 γ-secretase inhibitor (DAPT) for 48 h, and expression of AV canal and chamber markers was analysed with real time RT–PCR. Data were normalized to HPRT and expressed as folds of increase over untreated samples. ( g ) Untreated and DAPT-treated E9.5 hearts were subjected to ChIP assay analyses with anti-H3K27ac antibody. Pulled-down DNA fragments were analysed with RT–PCR and enrichment indicates the ratio of ChIPed DNA to negative control regions, normalized for input DNA. ( h ) Cartoon depicting the overlapping expressions of Hey1, 2 and Gata4 at stage E9.5–E10.5. Full size image Several lines of evidence suggest that the Notch target genes Hey1 and 2 could mediate the Gata4 dependent repression in the chambers. First, Hey1 and 2 factors have been shown to act as transcriptional repressors by recruiting Hdac1 (ref. 39 ). Second, although the regulatory sequences of cGata6 , Cx30.2 and cTnI do not contain consensus Hey-binding sites (that is, E-box), it has been reported that Hey factors can mediate repression via the interaction with GATA factors [39] , [40] . Moreover, Hey1 and 2 are selectively expressed in atrial and ventricular myocardium, respectively, but not in AV myocardium, and were shown to be involved in boundary formation between the AV canal and the chambers [41] , [42] . Analysis of Hey2 ChIP-seq data performed in mouse ESC revealed that the regulatory regions of Tbx2 , Cx30.2 and cTnI are occupied by Hey2 ( Fig. 1i and Supplementary Fig. 2 ). When co-transfected, Hey1 or Hey2 suppressed the Gata4-Smad-mediated activation of the AV canal enhancers in cell culture ( Fig. 4e ). To determine whether these AV canal enhancers were regulated by Notch target genes in vivo , cultured chambers from E9.5 Tbx3BAC-GFP; NppbBAC-Katushka mouse embryonic hearts were treated with the Notch inhibitor DAPT ( Fig. 4f ). The expression of marker of AV canal ( Tbx2 , Tbx3 ) increased ( Fig. 4f ). This was associated with an enrichment of the H3K27ac epigenetic mark on AV canal-specific enhancers ( Fig. 4g ). We conclude that these Gata4 responsive enhancers are suppressed in the chambers in response to Notch signalling ( Fig. 4h ). Compartment-specific co-factors function via GATA sites To assess whether the GATA sites are necessary for recruiting activators and repressors, we mutated the three GATA sites in the cGata6 enhancer and the two GATA sites in the Tbx2 enhancer ( Fig. 5a,b ). Mutation of the GATA sites affected the activation of the mutated enhancers by Gata4 ( Fig. 5a ). The increase in activity by addition of TSA was lost for the mutated enhancers ( Fig. 5a ). The co-activation of these mutated enhancers by Gata4 and Bmp2 effectors was significantly reduced ( Fig. 5b ). To assess whether the GATA sites are sufficient for recruiting activators and repressors, eight copies of the mutated 47 bp cGata6 enhancer module (cGata6muSP(GATA) 16 ) were coupled to a luciferase reporter ( Fig. 5c ). Similarly to the wild-type 102 bp enhancer, the cGata6muSP(GATA) 16 module was activated ~100-fold by Bmp2 effectors and Gata4, indicating that the preserved GATA sites are sufficient for the synergistic activation by Gata4 and Bmp2 effectors. When Hey1 or Hey2 where co-transfected, a significant inhibition of the stimulated reporter activity was observed. Similarly, HDAC1 and 2 were able to suppress the synergistic activation by Gata4 and Bmp effectors. These data are consistent with a model in which GATA sites serve as a platform to recruit co-factors that, in turn, mediate gene activation or repression, thus allowing GATA site-containing AV canal enhancers to act as tissue-specific transcriptional switches ( Fig. 5d ). 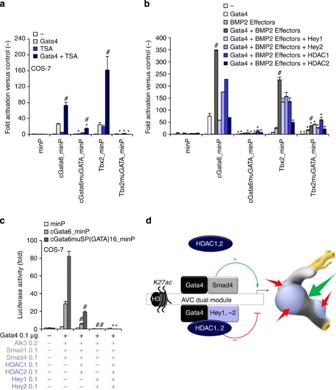Figure 5: GATA sites serve as a scaffold to recruit functionally distinct complexes. (a,b)In vitroreporter assays with thecGata6(102 bp) andTbx2(380 bp) luciferase constructs containing mutations for GATA sites (cGata6muGATA, Tbx2muGATA). Cos-7 cells co-transfected with Gata4, Alk3CA, Smad1 and 4, Hey1, 2, HDAC1 and 2 expressing vectors or not were treated in the absence or presence of 30 nmol l−1TSA (mean±s.e.m.,n=3,#P<0.05 for Gata4 or TSA/BMP2 treatment versus Gata, TSA or BMP2 alone, *P<0.05 for mutated versus wild-type enhancers using two- and three-way analysis of variance (ANOVA)). (c)In vitroreporter assays on 102 bpcGata6and mutated 47 bpcGata6enhancer (cGata6muSP). Cos-7 cells were co-transfected with Gata4 and Gata4 co-activators and co-repressors (mean±s.e.m.;n=3;#P<0.05 for HDAC1, 2 or Hey1, 2 versus Gata4 and BMP2 effectors; *P<0.05 for HDAC1, 2 and Hey1, 2 versus HDAC1, 2.$P<0.05 for HDAC1, 2 and Hey1, 2 versus Hey1, 2 using three-way ANOVA. (d) GATA-binding site-enhancers recruit a Gata4/Smad4/Hat transcriptional activation complex in the AV canal and a Gata4/Hey1,2/Hdac transcriptional repression complex in the chambers, which coordinately establish AV canal gene specificity. Figure 5: GATA sites serve as a scaffold to recruit functionally distinct complexes. ( a , b ) In vitro reporter assays with the cGata6 (102 bp) and Tbx2 (380 bp) luciferase constructs containing mutations for GATA sites ( cGata6muGATA, Tbx2muGATA ). Cos-7 cells co-transfected with Gata4, Alk3CA, Smad1 and 4, Hey1, 2, HDAC1 and 2 expressing vectors or not were treated in the absence or presence of 30 nmol l −1 TSA (mean±s.e.m., n =3, # P <0.05 for Gata4 or TSA/BMP2 treatment versus Gata, TSA or BMP2 alone, * P <0.05 for mutated versus wild-type enhancers using two- and three-way analysis of variance (ANOVA)). ( c ) In vitro reporter assays on 102 bp cGata6 and mutated 47 bp cGata6 enhancer ( cGata6muSP ). Cos-7 cells were co-transfected with Gata4 and Gata4 co-activators and co-repressors (mean±s.e.m. ; n =3; # P <0.05 for HDAC1, 2 or Hey1, 2 versus Gata4 and BMP2 effectors; * P <0.05 for HDAC1, 2 and Hey1, 2 versus HDAC1, 2. $ P <0.05 for HDAC1, 2 and Hey1, 2 versus Hey1, 2 using three-way ANOVA. ( d ) GATA-binding site-enhancers recruit a Gata4/Smad4/Hat transcriptional activation complex in the AV canal and a Gata4/Hey1,2/Hdac transcriptional repression complex in the chambers, which coordinately establish AV canal gene specificity. Full size image We found that enhancers that mediate AV canal-specific gene activity are activated in the AV canal myocardium and repressed in chamber myocardium, thus acting as tissue-specific switches. Histone H3K27 acetylation marks active enhancers [21] . Although the pattern of this modification has been assessed genome-wide in heart tissue by ChIP-sequencing [24] , the data do not provide cell type- or cardiac compartment-specific information (whole hearts were analysed, the heart contains many fibroblasts and other cell types). We assessed the genome-wide H3K27ac pattern in isolated embryonic AV canal and in chamber cardiomyocytes, respectively, and found prominent compartment-specific H3K27ac patterns. Specifically, we observed that most of the established AV canal-specific loci were strictly associated with H3K27ac in the EGFP-labelled AV canal cells. Conversely, except for firmly established chamber loci such as Nppa , Nppb and Hey2 , we found very few loci that were strictly enriched in H3K27ac in the Katushka-labelled chamber cells. Therefore, our data implicate this epigenetic signature in the regulation of embryonic AV canal specificity. The AV canal enhancers appeared to function through GATA factor-binding sites that are required and largely sufficient for both activation and repression functions. Mutation of GATA-binding sites with confirmed Gata4 occupancy, abolished activating and repressive activities, and a minimal enhancer module in which only GATA sites were maintained was sufficient to suppress activity in the chambers. We therefore identified a class of AV canal-specific enhancers essentially composed of GATA-binding sites and marked by AV canal-specific H3K27ac. Although the genome contains thousands of occupied GATA sites, it is not clear why only a fraction of these sites have AV canal-specific properties. We therefore assume that AV enhancers contain unidentified binding sites for additional factors that specify GATA site-dependent complex recruitment to drive AV canal-specific gene expression. Gata4 and Gata6 are essential for cardiogenesis. They are co-expressed in the myocardium and function redundantly [43] . Focusing on Gata4, we observed its presence in the nuclei of both AV canal and chambers coinciding with enhancer occupancy in both these compartments. Therefore, we explored the possibility of the presence of compartment-specific co-factors to try and explain the spatial restriction of AV canal enhancer activity. Bmp2, an AV canal-specific Bmp ligand, is required for AV canal-specific gene expression, although the mechanism of enhancer activation has not been established [13] , [26] , [44] , [45] . We observed that Smads (Smad4, Smad1/5), downstream effectors of Bmp2 (ref. 46 ), strongly activate the enhancers in a Gata4 and GATA-binding site-dependent manner. The in vivo H3K27ac ChIP data support a mechanism in which the activating Gata4/Smad complex recruits Hats such as p300 to a specific subset of AV regulatory regions, thereby inducing H3K27 acetylation and activation of AV canal genes. We identified a novel repressive mode of AV canal enhancers in the chamber myocardium, which restricts their activity to the AV canal. This observation suggests that, in addition to the localized Bmp2-mediated activation mechanism, an additional layer of regulation is involved in limiting enhancer activity to the AV canal. One of the AV canal enhancers studied in this respect regulates Tbx2, a T-box factor critical for AV canal development. This factor effectively blocks chamber differentiation [10] , [47] , [48] , [49] , indicating that delimiting its activity to the AV canal is critical for establishing correctly localized AV canal development. The transcription factors that activate cardiac and AV canal enhancers are typically expressed in both AV canal and chamber myocardium ( Supplementary Table 1 ). Furthermore, non-Bmp2-mediated Bmp-signalling is present in the chamber myocardium. Loss of function of Bmp6, -7 and -10, BmpR1A (Alk3) and Smad4 results in chamber and septal defects [50] , [51] , [52] , [53] , [54] . The repressive activity in chamber myocardium we identified may therefore be required to suppress activation of AV canal-specific enhancers in the chambers by these spatially less unrestricted activators. Our results indicate that in chamber myocardium, Gata4 cooperates with Hdac1 and 2 and induces H3K27 deacetylation of AV canal gene loci, providing the context for repressing gene activity. Whether, and to what extent, this repression is chamber-specific, is not clear. None of the Hdacs examined showed any specificity for chamber myocardium. Furthermore, Hdac1 and 2 were localized in the nuclei of both AV canal and chamber myocardium ( Fig. 4 ), and therefore are available for their deacetylation and repression functions. Our data suggest that Hey1 and Hey2, expressed in atrial chamber and ventricular chamber myocardium, respectively [41] and able to interact with Gata4 (ref. 40 ) and thus provide chamber-specificity to the Gata–Hdac activity. Furthermore, we identified a common, AV canal cell type-specific chromatin signature for AV canal-specific loci, which includes H3K27ac and co-occupancy of Gata4, Smad4 and Hey2 proteins. Previous work demonstrated that deficiency of both Hey1 and 2 results in moderate expansion of Tbx2 expression in the chambers [41] , [55] , suggesting that these factors contribute, but are not solely responsible for chamber repression by Gata4-Hdac. Previous work revealed that chromatin remodelling enzymes regulate Gata4 target genes by post-translational modifications of Gata4 (ref. 20 ). Gata4 was found to interact with Hdac2 and Hopx, a homeodomain-only protein required for heart development [37] . In the adult heart, Hopx is enriched in and required for the function of the AV conduction system [56] . Hdac2-mediated deacetylation of Gata4 may result in repression of Gata4 target genes in the AV canal and the derivative tissues. The PRC2 complex, a critical repressor required for normal lineage-specific differentiation, methylates Gata4, attenuating its transcriptional activity by reducing its interaction with and acetylation by p300 (ref. 57 ). Currently, we do not have data regarding the compartment specificity of such post-translational modification activities that could contribute to the spatial activity of the GATA-binding site-dependent AV canal enhancers. However, we hypothesize that the Gata4-Smad-HAT complex present in the AV canal would effectively compete with this mechanism and result in the activation of GATA site-dependent AV canal enhancers ( Fig. 5d ). The AV canal myocardium is a central component of the cardiac conduction system in vertebrates [58] , [59] . It has pacemaker properties and its gene expression profile is distinct from that of the chamber myocardium [58] , [59] . These properties are reminiscent of those of the embryonic heart tube, implicating that the mechanism dictating AV canal specificity is also active in the embryonic heart tube prior to the development of the chambers, but is repressed in the differentiating chamber cardiomyocytes [58] , [59] . Indeed, the cGata6 enhancer in mouse and bmp4 and tbx2b in zebrafish are active in the embryonic heart tube and maintain their primary, AV canal specificity by preventing their activity in the developing chambers, strikingly illustrating this process [44] , [60] , [61] . Confining this gene programme to the AV canal may be essential for the electrophysiological integrity of the heart. Mutations in Gata4 and Gata6 are responsible for congenital heart defects including AV canal defects and arrhythmias in humans and mouse models [14] , [20] , [62] , [63] , implicating their function in both chamber and conduction system tissues. Inactivation of both Hdac1 and 2 in the heart resulted in neonatal lethality associated with cardiac arrhythmias [35] . Interestingly, expression of conduction system genes Tnni1 , Cacna2d2 and Cacna1h [64] was upregulated in the heart chambers of Hdac1 and 2 double mutant mice [35] . Moreover, a regulatory region of the pacemaker channel Hcn4, active in pacemaker cells of the conduction system, was ectopically activated in the chambers by Hdac inhibition [65] . The broadly expressed factor Prox1 recruits Hdac3 and negatively regulates Nkx2.5 to ensure the functional and structural integrity of the pacemaker function in adult mice [66] . The Prox1-Hdac3-Nkx2.5 pathway appeared to be Hdac2 independent in cells [66] . This highlights the important role of Hdacs and chromatin-mediated mechanisms in the patterning of the AV conduction system. Our data suggest that Gata4-Hdac-mediated deacetylation of H3K27 serves as a mode of confinement of the conduction system gene programme, preventing its activity in the chambers. Dysfunction of this mechanism may result in misexpression of pacemaker genes in the chambers, resulting in arrhythmias. Ethics statement All animal work conformed to ethical guidelines and was approved by the animal ethical committee of the Academic Medical Center of Amsterdam. Transgenic reporter assay Each multimer of AV canal enhancer fragments was built in a geometric progression by first cloning a unit length PCR fragment, or annealed oligonucleotides in the case of the 47 bp and 102 bp cGata6 fragments, with SalI/XhoI ends into a similarly digested plasmid. Tetramers of the 380 bp ( Tbx2 ), 102 bp and 47 bp ( cGata6 ) fragments were released with SalI/XhoI, blunt-ended with Klenow and cloned into the SmaI site upstream of the promoter in the cTnT-lacZ construct. Tbx2muGATA-cTnT is identical to the Tbx2-cTnT construct, with the exception of 4-bp substitutional mutations of the GATA sites located at position −2312 and position −2345 of the Tbx2 enhancer region. (GATA, CAAGGATATTCT, GGTCGATAAAGA; GATAmu, CAAGTTTTTTCT, GGTCTTTTAAGA). The mutations were generated using the QuickChangeTM Site-Directed Mutagenesis kit (Stratagene). Tandemly repeated copies of a 102 bp cGata6 enhancer fragment were cloned into the hsp68-lacZ reporter vector as previously described. DNA was injected into the pronucleus of 0.5-day-old fertilized FVB/N eggs, which were subsequently transferred into the oviducts of CD-1 pseudopregnant foster females (Cyagen). At least 200 injections were performed per construct. Embryos were harvested and stained with X-gal to detect lacZ activity, and yolk sacs were processed for PCR genotyping. Only patterns that were observed in at least three different embryos resulting from independent transgenic integration events of the same construct were considered reproducible. A transgenic mouse line harbouring a BAC of the Nppb locus modified with the red fluorescent protein Katushka [23] was bred with a transgenic mouse line harbouring a BAC of the Tbx3 locus modified with the EGFP [19] . Embryonic explant culture Mouse E9.5 embryonic hearts explants, dissected in Dulbecco's modified Eagle's medium (DMEM), were cultured in DMEM supplemented with 5% fetal calf serum and penicillin/streptomycin for 48 h at 37 °C in 5% CO 2 . Trichostatin-A (Sigma), BMP2 (R&D Systems), Inhibitor IX (Calbiochem) or dimethylsulphoxide alone was added. Cell sorting E10.5 double transgenic hearts were dissected, pooled and digested with 0.25% Trypsin/EDTA (Invitrogen), neutralized in DMEM (Invitrogen) containing 5% FBS and 10 mmol l −1 HEPES (Invitrogen), rinsed and resuspended in phosphate-buffered saline (PBS) and passed through a 70-mm nylon cell strainer (Falcon). Samples were sorted on a FacsAria flow cytometer (BD) using Influx software. Samples were gated to exclude debris and cell clumps. The number of E10.5 AV canal GFP cells and chambers–Katushka cells per embryo obtained were typically 600–900 and 2,400–3,600, respectively. Fluorescent cells were collected into PBS and processed for RNA extraction or ChIP-seq. RNA isolation and real time RT–PCR Total RNA was isolated from treated explants and sorted cells with NucleoSpin RNA XS (Bioke) following the protocol of the manufacturer. cDNA was generated using Superscript II (Invitrogen) and OligodT as primers. Expression level of different genes was assessed with quantitative RT–PCR using the LightCycler Real-Time PCR system (Roche Diagnostics) and the primers described in Supplementary Table 4 . Values were normalized to HPRT expression levels. Chromatin immunoprecipitation E10.5 embryos were dissected, and the primary myocardium (AV canal/outflow tract) and atria and ventricle regions were separately collected in cold PBS. ChIP was performed with a True MicroChIP kit (Diagenode) according to the manufacturer’s protocol. Antibodies used for ChIP were anti-Gata4 (2 μg, Santa Cruz Biotechnology), anti-Smad4 (2 μg, Santa Cruz Biotechnology) and anti-H3K27ac (0.5 μg, Abcam ab4729). Chipped DNA were subjected to library preparation using the 5500 Series SOLiD Systems preparation kit (Applied Biosystems) according to manufactures recommendations and sequenced using the 5500 wildfire sequencer (SOLiD). Quantitative PCR was performed on a Roche LightCycler 480 System using Sybr Green detection. Fold enrichment indicates the ratio of ChIPed DNA to negative control regions, normalized for input DNA. Primer sequences are provided in Supplementary Information . Hey2 ChIP was performed in CM7/1 mouse ESC with doxycycline-inducible Flag-Hey2 expression [55] . 10^8 cells were induced with 50 ng μl −1 doxycycline for 48 h and ChIP was performed with an anti-Flag-M2 antibody (10 μg Sigma-Aldrich). Chipped DNA were subjected to library preparation using the NEBNext ChIP-seq sample preparation kit (New England Biolabs) according to manufacturer’s recommendations and sequenced on a GAIIx platform (Illumina). X-gal staining and immunohistochemistry For X-gal staining, embryonic hearts were dissected in PBS and then fixed for 10 min with 4% (wt/vol) paraformaldehyde in PBS. Embryos were washed twice with PBS and then stained with X-gal (Invitrogen) for 4–16 h at 37 °C. After developing the blue colour, embryos were rinsed in PBS and post-fixed in 4% (wt/vol) paraformaldehyde. Fluorescent immunohistochemistry on sections was carried out with anti-Gata4 (1:50, Santa Cruz Biotechnology), anti-cTnI (Millipore), anti-Hdac1 (1:200, Biovision) and anti-Hdac2 (1:200, Biovision) antibodies. Images were obtained with Leica DFC320 and Leica DM6000. In vitro and ex vivo reporter assays Tandemly repeated AV canal enhancers were cloned in pGL4-2.6-luciferase construct that contains a minimal promoter (Promega). Luciferase reporter constructs were co-transfected with expression constructs for human Gata4 (pcDNA3 [13] ), mouse Smad1 (pcDNA3 [13] ), Smad4 (pcDNA3 [13] ), constitutively active Bmp-receptor Alk3 (Alk3CA) (pCS2.BmpR1a.CA), Hey1, 2, HDAC1 and 2. Full-length mouse FLAG- Hey1, 2 were kindly provided by Dr Esther Creemers (Academic Medical Center, Amsterdam, the Netherlands). Full-length human HDAC2 was kindly provided by Dr John Epstein. Full-length human HDAC1 was purchased from Open Biosystem. Constructs were transfected into Cos-7 cells with the PEI transfection reagent. Cell extracts and luciferase assays were performed following the protocol of the manufacturer (Promega). The mean luciferase activities and standard deviations (s.d.) were plotted as fold activation when compared with the empty expression plasmid. For DNA transfection of AV canal explants, 50 ng of firefly luciferase reporter vector was mixed with 80 ng μg −1 of CMV β-galactosidase plasmid in 5 μl of OPTIMEM (Invitrogen); 0.5 μl of Lipofectamine 2000 (Invitrogen) was added to 5 μl of OPTIMEM. After 5 min, the DNA and Lipofectamine solutions were mixed together. After incubation for 20 min, the transfection reagent mixture (10 μl) was transferred into a well of a 384-well plate containing the explant in medium. Transfection assays were performed in quadruplo and the efficiency was assessed by the expression of a CMV-EGFP reporter. Explants were harvested 48 h after transfection and processed for chemiluminescence activity using the Dual-Light luminescent reporter gene assay (Invitrogen). Processing of ChIP-sequencing data and statistical analysis ChIP- seq data for H3K27ac in chamber-Katushka/AV canal-EGFP-sorted cells chamber-Katushka/AV canal-EGFP was processed using an in-house peak calling algorithm dubbed OccuPeak (van Duijvenboden et al. , submitted). Using an identical threshold ( P =0.01), peak calling resulted in 87,572 and 67,092 H3K27ac peaks in AV canal and chamber tissue, respectively. Microarray data [19] was used to determine a top-50 of AV canal-enriched genes ( Supplementary Tables 1,2 ). In addition, a custom list of firmly established AV canal-restricted genes was used ( Supplementary Tables 1,2 ). The coordinates of these genes were imported from the UCSC gene database. Gene regulation by H3K27 acetylation is expected to occur on both promoters and distal enhancers. Therefore, we defined gene loci as UCSC genes plus flanking regions of 50 Kb on either side. Peaks were considered to occupy a gene locus if they overlap it with 1 bp or more. Overlap was established using the Galaxy intersect tool ( https://www.main.g2.bx.psu.edu/ ). Compared with the chamber H3K27ac ChIP-seq data, the AV canal data contained 1.4 times the number of mapped reads. Therefore, we assumed that the difference in total number of ChIP-seq peaks called between AV canal- (87,572) and chamber tissue (67,092) does not reflect biology, but is caused by a difference in peak calling power between the data sets. To correct for this difference, we determined the number of peaks from both data sets as present in 5,541 random gene loci. This resulted in a 0 hypothesis in which AV canal peaks are 1.08 times more common than chamber peaks ( Supplementary Table 2 ). We assumed a normal distribution of H3K27ac ChIP-seq peaks across gene loci. The λ 2 test was used to analyse the frequency of H3K27ac peaks according to tissue type and gene cluster. Statistical significance was set at P <0.05. Occurrence of specific motifs among the Gata4 peaks was performed with MEME [67] . Biological process terms were identified using the DAVID informatics resource gene ontology analysis software [68] . Statistical analysis For gene expression analysis and ChIP assay, P- values were generated using the Student’s two-tailed t -test. For luciferase assays analysis of variance was used. Statistical significance was considered for P <0.05. Accession codes : Sequencing data have been deposited in Gene Expression Omnibus under accession number GSE55611 . How to cite this article : Stefanovic, S. et al. GATA-dependent regulatory switches establish atrioventricular canal specificity during heart development. Nat. Commun. 5:3680 doi: 10.1038/ncomms4680 (2014).